Improving the stability and optical properties of germanane via one-step covalent methyl-termination Two-dimensional van der Waals materials have shown great promise for a variety of electronic, optoelectronic, sensing and energy conversion applications. Since almost every atom in these two-dimensional crystals is exposed to the surface, covalent surface termination could provide a powerful method for the controlled tuning of material properties. Here we demonstrate a facile, one-step metathesis approach that directly converts CaGe 2 crystals into mm-sized crystals of methyl-terminated germanane (GeCH 3 ). Replacing –H termination in GeH with –CH 3 increases the band gap by ~0.1 eV to 1.7 eV, and produces band edge fluorescence with a quantum yield of ~0.2%, with little dependence on layer thickness. Furthermore, the thermal stability of GeCH 3 has been increased to 250 °C compared with 75 °C for GeH. This one-step metathesis approach should be applicable for accessing new families of two-dimensional van der Waals lattices that feature precise organic terminations and with enhanced optoelectronic properties. There has been remarkable widespread interest in the exploration of the unique properties and applications of single and few-layer thick sheets of layered van der Waals materials such as graphene or the layered transition metal dichalcogenides [1] , [2] , [3] , [4] , [5] , [6] , [7] . This work has shown the significant role of the immediate environment on the properties and reactivity of these van der Waals layers [8] . This suggests, on the other hand, the intriguing possibility of manipulating the properties of single-atom thick materials by covalent termination with rationally designed substituents. In contrast to the negligible role the surface binding ligand plays in nanoscale materials, terminating the surface of single-atom thick materials with different ligands is predicted to allow for the broad tuning of properties including band gap, band alignment, thermal stability, carrier mobility and spin-dependent interactions [9] , [10] . For example, a quantum spin Hall state with a surface-tunable spin-orbit gap has been recently predicted for two-dimensional (2D) Sn graphene analogues that are terminated with halides but not with hydrogen [11] , opening the door for novel lateral heterostructures between topological and conventional states. Unfortunately, most of the 2D materials studied to date comprise neutral van der Waals layers that lack the possibility of covalent functionalization. Although the functionalization of graphene with organic components, hydrogen atoms or even halogens have been achieved, these modifications completely disrupt the excellent electronic mobility of the Fermi–Dirac state, to produce 3–5 eV band gap semiconductors [12] , [13] , [14] , [15] . Researchers have recently developed layered van der Waals systems in which each surface atom requires a covalent ligand to become coordinatively saturated, such as the metal carbide/nitride MXenes, the amine coordinated II–VI chalcogenides, and the group IV graphene analogues such as silicane or germanane [9] , [16] , [17] , [18] , [19] , [20] . Because the valence/conduction bands of these materials are comprised of metal–metal or metal–anion bonding within the 2D plane [21] , rather than the π-bands such as that in graphene, these systems offer the possibility to tune the entire electronic properties on the basis of the identity and electron withdrawing capability of the substituent, without completely disrupting the relevant electronic states. The creation of many of these surface-terminated layered materials often relies on topotactic methods to interconvert a precursor layered crystal structure directly into the van der Waals material, frequently through deintercalation in acidic aqueous conditions that can result in partial surface termination with unwanted oxide or hydroxide states. For example, the deintercalation of layered Zintl phases, such as CaSi 2 in aqueous HCl produces the air and water reactive, partially hydroxide-terminated silicane SiH x (OH) 1−x as evidenced by the existence of broad Si-O stretches that occur between 1,000–1,200 cm −1 in the Fourier Transform Infrared (FTIR) spectrum [19] , [20] . This ambiguity in surface functionalization convolutes efforts to correlate the effects of surface functionalization on the optoelectronic properties of these single-atom thick semiconductors [9] , [20] , [22] , [23] , [24] . Furthermore, it is well established that H-terminated Si(111) and Ge(111) surfaces are extremely air reactive, whereas the –CH 3 terminated surfaces can be resilient towards oxidation [25] , [26] . To bypass the potential air-reactive intermediates and create new organic-terminated materials, new single-step synthetic methods that can directly convert a precursor crystalline solid-state crystal into a crystalline, exfoliatable, organic-terminated van der Waals solid in nonaqueous solvents is required. Towards these ends, we report a one-step metathesis approach that directly converts CaGe 2 into GeCH 3 , a methyl-terminated layered van der Waals solid. Structural characterization The crystal structure of CaGe 2 consists of hexagonal, puckered sp 3 layers of Ge − atoms that are separated by Ca 2+ ions ( Fig. 1a ). We hypothesized that the anionic Ge − on the surface and edges of the crystals could react topotactically in an S N 2 or metathesis-like fashion with a small organic molecule, such as CH 3 I, to form a Ge–CH 3 bond along with CaI 2 . The expansion of the lattice would allow the precursors to diffuse inward and the reaction would proceed to completion. However, in our initial experiments with pure CH 3 I, only the surface layers of CaGe 2 had reacted, likely due to the low solubility of CaI 2 . Instead, we developed a biphasic CH 3 I/H 2 O solvent reaction in which 2–3 mm crystals of CaGe 2 are fully immersed in CH 3 I, while CaI 2 is transferred into the H 2 O layer ( Supplementary Fig. 1 ). After rinsing in concentrated HCl to remove any trace residual CaI 2 , and then isopropanol, the reaction yields crystals of GeCH 3 that are ~1 mm in diameter and <100 μm in thickness ( Fig. 1b and Supplementary Fig. 2 ). Single-crystal X-ray diffraction (XRD) analysis ( Fig. 1c ) shows that each one of these crystallites is a single crystal having a hexagonal spacing of a =3.96 Å; however, the interlayer turbostratic disorder and curvature of these crystallites preclude determination of the c axis spacing. Powder XRD analysis ( Fig. 1d ) of GeCH 3 confirms that it can be fit to a 2H unit cell (two GeCH 3 layers per hexagonal unit cell spacing) with a =3.97 Å and c =17.26 Å (8.63 Å per layer). This corresponds to a 0.09 Å expansion in the a -direction and a 3.1 Å increase per layer compared to GeH, which has lattice parameters of a =3.880 Å and c =11.04 Å (5.50 Å per layer) [9] . This 3.1 Å increase is close to twice the difference between the Ge–C bond length (1.95 Å) and the Ge–H bond length (1.52 Å) plus twice the difference between the van der Waals radii of –CH 3 (2.0 Å) and –H (1.2 Å), further indicating substitution of the –H substituent with a –CH 3 substituent ( Supplementary Fig. 3 ). 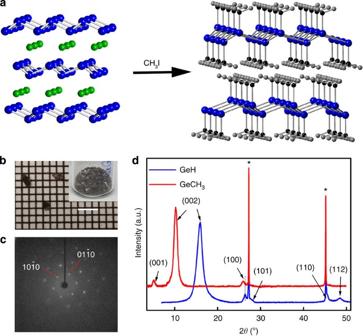Figure 1: The one-step topotactic transformation of CaGe2into GeCH3crystals. (a) Schematic illustration of conversion of CaGe2(left) into GeCH3(right). (b) Optical images of GeCH3crystals with select crystals on graph paper with a 1 mm grid. Scale bar, 3 mm. (c) Single-crystal XRD pattern of GeCH3collected down the [001] zone axis. (d) Powder XRD patterns of GeH (blue) and GeCH3(red). The starred peaks correspond to diffraction reflections of an internal Ge standard. The dotted line highlights the changes in the 100 reflections between GeH and GeCH3. XRD, X-ray diffraction. Figure 1: The one-step topotactic transformation of CaGe 2 into GeCH 3 crystals. ( a ) Schematic illustration of conversion of CaGe 2 (left) into GeCH 3 (right). ( b ) Optical images of GeCH 3 crystals with select crystals on graph paper with a 1 mm grid. Scale bar, 3 mm. ( c ) Single-crystal XRD pattern of GeCH 3 collected down the [001] zone axis. ( d ) Powder XRD patterns of GeH (blue) and GeCH 3 (red). The starred peaks correspond to diffraction reflections of an internal Ge standard. The dotted line highlights the changes in the 100 reflections between GeH and GeCH 3 . XRD, X-ray diffraction. Full size image Transmission-mode Fourier Transform Infrared spectroscopy further confirms the –CH 3 surface termination in GeCH 3 ( Fig. 2a ) and that our sample is free of residual oxide. In GeCH 3 , the major Ge–H stretching frequency [9] , [24] , [27] , [28] , [29] at ~2,000 cm −1 is almost completely gone and replaced by a Ge–C stretch [29] that occurs at 573 cm −1 . The other major modes that are observed in GeCH 3 correspond to –CH 3 stretching at 2,907 and 2,974 cm −1 , –CH 3 bending at 1,403 and 1,237 cm −1 and –CH 3 rocking at 778 cm −1 (refs 29 , 30 ). The residual amount of Ge–H stretching suggests that there exists a small percentage of –H termination, and elemental analysis suggests that 90%±10% of the Germanium atoms are terminated with –CH 3 . This residual –H could result either from the minor solubility of H 2 O in CH 3 I, or during the washing process. To further confirm the identity of each vibrational mode, we also created Ge 13 CH 3 and GeCD 3 . In Ge 13 CH 3 , the Ge–C stretch shifts down to 558 cm −1 , and the other –CH 3 vibrational modes slightly decrease by 1–10 cm −1 ( Supplementary Table 1 ). There is a much more significant change in the vibrational energies of GeCD 3 , as the –CD 3 stretching modes are shifted to 2,240 and 2,116 cm −1 , the –CD 3 bending mode decreases to 1,024 and 954 cm −1 , the –CD 3 rocking mode decreases to 584 cm −1 , and the Ge–CD 3 stretch decreases to 530 cm −1 ( Supplementary Table 1 ) [29] . As the 778 cm −1 CH 3 rocking mode can possibly mask the existence of any residual Ge–O–Ge or Ge–O vibrational modes which normally occur from 800–1,000 cm −1 (refs 24 , 28 ), the shift of this rocking mode in GeCD 3 allows elucidation of any residual Ge–O–Ge or Ge–O. The only vibrational modes observed in this region for GeCD 3 are the 770 and 830 cm −1 vibrations that correspond to bond-bending Ge–H 2 modes from nearest neighbour Ge atoms at the crystal edges [9] , [27] , [28] . X-ray Photoelectron Spectroscopy (XPS) measurements indicate a single Germanium +1 oxidation state ( Fig. 2b ), further suggesting that GeO 2 and other surface oxides are not present. The Ge 2p 3/2 peak occurs at 1,217.5 eV, which is slightly shifted compared with the observed 1,217.8 eV peak of GeH, but consistent with CH 3 -terminated Ge(111). This slight shift to lower XPS binding energy is consistent with previously observed XPS spectra of –H or –CH 3 terminated silicon surfaces [25] . 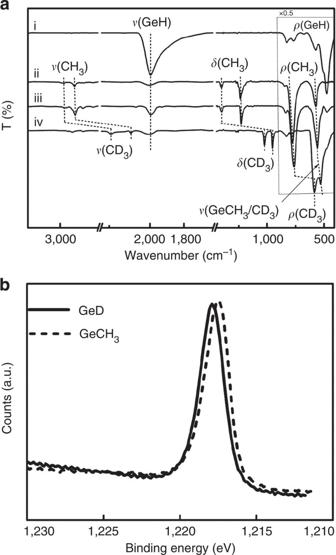Figure 2: The surface terminating chemistry of GeCH3. (a) FTIR spectra of GeH (i), GeCH3(ii), Ge13CH3(iii) and GeCD3(iv). The intensity of the four spectra are all multiplied by 0.5 in the range of 400–900 cm−1. (b) XPS spectra of the Ge 2p3/2peak for GeH (solid line) and GeCH3(dashed line), indicating exclusively Ge+1on the surface. XPS, X-ray photoelectron spectroscopy. Figure 2: The surface terminating chemistry of GeCH 3 . ( a ) FTIR spectra of GeH (i), GeCH 3 (ii), Ge 13 CH 3 (iii) and GeCD 3 (iv). The intensity of the four spectra are all multiplied by 0.5 in the range of 400–900 cm −1 . ( b ) XPS spectra of the Ge 2p 3/2 peak for GeH (solid line) and GeCH 3 (dashed line), indicating exclusively Ge +1 on the surface. XPS, X-ray photoelectron spectroscopy. Full size image Optical properties and band structure The absorption and fluorescence measurements of GeCH 3 are consistent with that of a direct band gap semiconductor. GeCH 3 has strong photoluminescence (PL) emission centred at 1.7 eV (730 nm (red)), which is close to the observed diffuse reflectance absorption (DRA) onset at 1.69 eV ( Fig. 3a ). This corresponds to a 0.1 eV increase in band edge compared with GeH (1.59 eV) ( Fig. 3b ). Band structure calculations for the measured structure using the hybrid HSE06 (refs 31 , 33 , 33 ) exchange-correlation functional, confirm this band gap, and predict that the two-layer unit cell has a direct band gap of 1.82 eV ( Fig. 3c ). The red PL can be easily detected by eye under UV illumination in both solid-state samples and in suspension in isopropanol ( Fig. 3d ). The full-width at half maximum of the fluorescence emission is ~250 meV. The absolute quantum yield of the solid flakes was measured to be 0.23%. This represents a minimum bound of the quantum yield, due to the difficulty in correcting for self-absorption in solid-state measurements. The full-width at half maximum and quantum yield values are close to those observed in exfoliated single-layer MoS 2 , which are 50–150 meV, and 0.4–0.5% [34] , [35] , respectively. We hypothesize that even further improvements in the quantum yield could arise with better control over the degree of –CH 3 versus –H functionalization. In MoS 2 and many other metal dichalcogenides, a direct band gap is only observed when exfoliated down to single layers [36] , making the preparation of large-area single layers a necessary and challenging requirement before optoelectronic devices can be fabricated. In contrast, we observe that the photoluminescence emission intensity of exfoliated samples is linearly proportional to the number of layers from 13–65 layers ( Fig. 3e and Supplementary Fig. 4 ). The band edge emission does not depend on layer thickness, at least with 13 layers and above, reflecting the relatively weak electronic coupling and orbital overlap of the conduction and valence bands in neighbouring layers. This is in contrast to the overlap of neighbouring C 2p z orbitals in graphite, as well as the S 3p z orbitals at the Γ point in MoS 2 (ref. 36 ). Finally, the intense PL contrasts with our observations on our previously reported crystals of GeH, of which we have yet to observe any band edge PL [9] . Taken together, this data shows that the nature of the covalently modifiable surface ligand can tune the optoelectronic properties of these materials. 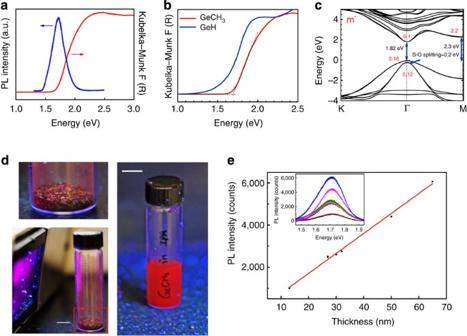Figure 3: The optical properties and band structure of GeCH3. (a) DRA (red) and PL (blue) of GeCH3. (b) DRA spectra of GeH (blue) and GeCH3(red) plotted in Kubelka-Munk function versus photon energy. (c) Electronic band structure of a bilayer GeCH3unit cell calculated using the hybrid HSE06 theory including spin-orbit coupling with experimental lattice parameters (3.96 Å) predicting a 1.82 eV direct band gap. The hole and electron effective masses for each extrema are indicated in red. (d) Images of GeCH3photoluminescence of crystals (left) and in suspension in isopropanol (right), upon illumination with a handheld 365 nm light. Scale bars, 1 cm. (e) PL intensity of exfoliated GeCH3thin flakes having average thicknesses ranging from 13–65 nm. Inset is the raw photoluminescence spectra of flakes with the thickness of 13 nm (wine), 27 nm (violet), 29 nm (orange), 31 nm (olive), 49 nm (magenta) and 65 nm (blue). Figure 3: The optical properties and band structure of GeCH 3 . ( a ) DRA (red) and PL (blue) of GeCH 3 . ( b ) DRA spectra of GeH (blue) and GeCH 3 (red) plotted in Kubelka-Munk function versus photon energy. ( c ) Electronic band structure of a bilayer GeCH 3 unit cell calculated using the hybrid HSE06 theory including spin-orbit coupling with experimental lattice parameters (3.96 Å) predicting a 1.82 eV direct band gap. The hole and electron effective masses for each extrema are indicated in red. ( d ) Images of GeCH 3 photoluminescence of crystals (left) and in suspension in isopropanol (right), upon illumination with a handheld 365 nm light. Scale bars, 1 cm. ( e ) PL intensity of exfoliated GeCH 3 thin flakes having average thicknesses ranging from 13–65 nm. Inset is the raw photoluminescence spectra of flakes with the thickness of 13 nm (wine), 27 nm (violet), 29 nm (orange), 31 nm (olive), 49 nm (magenta) and 65 nm (blue). Full size image Thermal stability We previously observed that GeH begins to amorphize upon annealing at 75 °C, is completely amorphous above 175 °C and starts to dehydrogenate between 200 °C and 250 °C [9] . In contrast, GeCH 3 has considerably enhanced thermal stability. According to thermogravimetric analysis, a transition occurs starting at 300 °C ( Fig. 4a ) that corresponds to the expected mass loss for approximately 90% CH 3 -termination, which is in excellent agreement with our elemental analysis. We have previously found that DRA is a much more sensitive probe of the degree of amorphization than any other technique, due to the reduced band gap of amorphous germanium [9] . There is virtually no shift in band edge emission up to 200 °C, whereas after annealing at 250 °C and 300 °C, the band edge red-shifts by 0.06 and 0.10 eV, respectively ( Fig. 4b ). The powder XRD pattern also shows negligible changes after annealing up to 250 °C, but it is almost completely amorphous after annealing at 300 °C ( Fig. 4c ). The intensity of photoluminescence emission also started to decrease after annealing at 250 °C ( Fig. 4d ). These techniques collectively demonstrate that GeCH 3 begins to amorphize at 250 °C. Considering the lack of any PL in our previous studies on GeH, the enhanced stability upon methyl-termination is likely necessary to realize semiconductor properties such as band edge photoluminescence that are often disrupted by defect states. 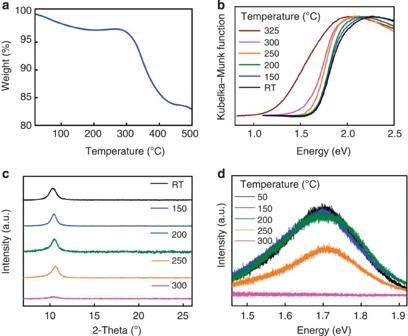Figure 4: The enhanced thermal stability of GeCH3. (a) Thermogravimetric analysis of GeCH3. (b,c) DRA spectra (b) and powder XRD patterns (c) of bulk GeCH3after annealing in 5% H2/Ar for four hours at various temperatures. (d) Photoluminescence spectra of a single exfoliated GeCH3flake using the same annealing procedure. Figure 4: The enhanced thermal stability of GeCH 3 . ( a ) Thermogravimetric analysis of GeCH 3 . ( b , c ) DRA spectra ( b ) and powder XRD patterns ( c ) of bulk GeCH 3 after annealing in 5% H 2 /Ar for four hours at various temperatures. ( d ) Photoluminescence spectra of a single exfoliated GeCH 3 flake using the same annealing procedure. Full size image In summary, we have created for the first time GeCH 3, a covalently modified direct band gap germanane, via a one-step topotactic metathesis reaction of CaGe 2 crystals with CH 3 I. We have shown that covalent methyl surface termination not only increases the band gap by 0.1 eV, but also enhances the thermal stability compared with GeH. The photoluminescence quantum yield is on the same order of magnitude as other single-layer metal chalcogenides, but does not have the stringent single-layer requirement to observe such band edge emission, making these materials intriguing building blocks for future optoelectronic devices. This topotactic metathesis reaction can be extended to create new families of organic-terminated van der Waals materials from other solid-state crystal structures. Dimensionally reduced atomic-scale derivatives can have dramatically different properties than their parent analogue, which can be tuned with the nature of the surface substituent. Synthesis To synthesize CaGe 2 crystals, Ca and Ge were loaded into a quartz tube with stoichiometric ratio. The quartz tube was sealed under vacuum and annealed at 950–1,050 °C for 16–20 h and then slowly cooled down to room temperature [9] . To synthesize GeCH 3 , the CaGe 2 crystals were loaded into an extraction thimble, fully immersed in iodomethane (Sigma Aldrich), with a separated distilled water phase outside in the beaker and stir bar at the bottom of the extraction thimble ( Supplementary Fig. 1 ). The reaction was running at room temperature for a week. Then the exfoliated flakes were rinsed with isopropanol (Sigma Aldrich), concentrated HCl(aq) (Fisher, Certified ACS Plus) followed by isopropanol. The sample was then dried on a Schlenk line at room temperature. For all thermal stability study experiments, the room temperature sample was annealed at different temperatures in flowing 5% H 2 in Ar, then cooled down and characterized at room temperature. Characterization Powder XRD (Bruker D8 powder X-ray diffractometer, Rigaku MiniFlexII X-Ray diffractometer) and Single-crystal XRD (Nonius Kappa CCD diffractometer) were used to study the structure of GeCH 3 . FTIR measurements were collected on a Perkin-Elmer Frontier Dual-Range FIR/MidIR spectrometer that was loaded in an Ar-filled glovebox. XPS was collected using a Kratos Axis Ultra X-ray photoelectron spectrometer equipped with a monochromated (Al) X-ray gun. The atomic force microscopy (AFM) images were collected on a Bruker AXS Dimension Icon Atomic/Magnetic Force Microscope with Scan Asyst. DRA measurements (Perkin-Elmer Lambda950 UV/Vis Spectrometer) and PL (Cary Eclipse Fluorescence Spectrophotometer) measurements were conducted to study the optical properties of the bulk solid crystals. In the PL measurements, the excitation wavelength was set to 380 nm, the excitation and emission slit widths were set to 20 nm and 5 nm, respectively. The absolute Quantum Yield of the solid samples was measured with the Quanta-phi (HORIBA Scientific) assembled in Fluorolog (HORIBA Scientific). The temperature-dependent and the thickness-dependent PL measurements were collected using a Renishaw InVia Raman equipped with a CCD detector upon excitation using a 633-nm HeNe laser at a power density of ~24 mW cm −2 , with a laser spot size of ~2 μm diameter. To collect the thickness-dependent measurement, we exfoliated GeCH 3 onto 285 nm SiO 2 /Si. The thicknesses of these flakes were measured by AFM to identify exfoliated flakes that had regions of relatively uniform thickness larger than the excitation spot size. The weighted average height from the AFM measurement was used to determine the thickness. For the temperature-dependent PL, exfoliated flakes were annealed at different temperatures in 5% H 2 /Ar, and their PL was recollected on the same flake after cooling down to room temperature. The same trend was observed for three different exfoliated flakes. Thermogravimetric Analysis (Q-500 thermogravimetric analyzer) was collected in flowing N 2 at 10 °C min −1 . Elemental Analysis (Atlantic Microlab Inc) of the C/H ratio was collected to determine the ratio of CH 3 -termination to H-termination. Exfoliation of GeCH 3 flakes To study the PL intensity of GeCH 3 flakes with different thickness. The bulk GeCH 3 flakes were exfoliated onto 285 nm SiO 2 /Si substrate with kapton tape. The tape residue was cleaned with acetone and then by isopropanol, followed by a N 2 blow dry to clean the residue solvent on the substrate. The thickness of these flakes was confirmed by AFM before the PL measurement. The AFM images are shown in Supplementary Fig. 4 , the colour of the dots in AFM height profiles corresponds to the colour of the PL spectra in Fig. 3e . Calculations Density functional theory calculations were performed using the Vienna Ab initio simulation package [37] , [38] . The effect of the core electrons was included using projector augmented wave pseudopotentials [39] . To simulate GeCH 3 monolayers, we used a supercell with a vacuum of 20 Å and with the in-plane lattice parameter fixed to the experimental value a =3.97 Å. Bilayer GeCH 3 was simulated using a supercell with lattice parameters fixed to a =3.97 Å and c =17.26 Å. Relaxation of the ionic positions was done using the Perdew–Burke–Ernzerhof exchange correlation functional [40] , [41] with a plane-wave cutoff energy of 600 eV and a 9 × 9 × 1 Monkhorst Pack k-point mesh [42] . To obtain an accurate description of the band gap, we performed high-level calculations based on the HSE06 hybrid functional [31] , [32] , [33] . How to cite this article: Jiang, S. et al. Improving the stability and optical properties of germanane via one-step covalent methyl-termination. Nat. Commun. 5:3389 doi: 10.1038/ncomms4389 (2014).